Wind direction and proximity to larval sites determines malaria risk in Kilifi District in Kenya Studies of the fine-scale spatial epidemiology of malaria consistently identify malaria hotspots, comprising clusters of homesteads at high transmission intensity. These hotspots sustain transmission, and may be targeted by malaria-control programmes. Here we describe the spatial relationship between the location of Anopheles larval sites and human malaria infection in a cohort study of 642 children, aged 1–10-years-old. Our data suggest that proximity to larval sites predict human malaria infection, when homesteads are upwind of larval sites, but not when homesteads are downwind of larval sites. We conclude that following oviposition, female Anophelines fly upwind in search for human hosts and, thus, malaria transmission may be disrupted by targeting vector larval sites in close proximity, and downwind to malaria hotspots. Malaria remains an important public health problem in disease endemic parts of sub-Saharan Africa [1] , where mosquitoes of the Anopheles gambiae complex are the main vectors of Plasmodium falciparum . Recent efforts to reduce the global malaria burden have led to the introduction of Artemisinin combination therapy as first-line anti-malarial treatment [2] , and improved coverage of populations at risk of infection with long-lasting insecticidal nets (LLINs), which reduce vector numbers and reduce the human-vector contact [3] . In association with these efforts, there have been reports of declining malaria cases and mortality in parts of Africa [4] , [5] , [6] , [7] , leading to renewed optimism towards the achievement of longer term malaria elimination and/or eradication. However, hotspots of malaria are widely observed [8] , [9] , [10] , and seem to persist in areas of falling transmission [11] . The effect of these hotspots is to make malaria more difficult to control [12] , [13] . However, to counter this effect, it is possible to target extra control measures on the hotspots. The anopheles mosquito life cycle and its interaction with malaria transmission is complex. To reproduce, female mosquitoes need to take a blood meal to nourish their eggs, and then oviposit in suitable water bodies. Mosquitoes may acquire malaria parasites during a blood meal. After several feeding cycles, the mature female mosquitoes may become infectious, and on biting a second human host may transmit malaria parasites. The dispersion distance of adult mosquitoes is limited, and includes a fitness cost [14] . The proximity of host and larval sites will therefore determine mosquito dispersion and survival. Thus, the heterogeneous spatial distributions of larval sites and human hosts are expected to lead to intermediate heterogenous spatial distributions of biting [15] . It is well known that malaria risk can be predicted by the proximity of a human residence to geographical features associated with larval sites [16] , [17] . Vector control measures are likely to be more effective if intensified on hotspots [18] . The relationship between fine scale heterogeneity of transmission and larval sites has not been explored. Furthermore, although models have examined the relationship between heterogeneous populations and heterogeneous biting, there are few epidemiological data to examine how mosquito ecology and searching for human hosts and larval sites leads to hotspots [15] . In this study, we explore the association during a single rainy season between the spatial distribution of febrile and asymptomatic malaria in children and the location of Anopheles larval sites and local geographical features in a rural area of Kilifi District on the Kenyan coast. Malaria is endemic with peaks of disease incidence occurring shortly after the rainy season. A. gambiae s.l. has the major role in malaria transmission [19] . Anopheles funestus has also been found in Kilifi District, and other species such as Anopheles nili and Anopheles moucheti may be present, but have not been frequently identified [20] . The study area and malaria incidence The study area covered 40 square kilometres (10 km North to South and 4 km East to West). We enrolled 642 children within the study area, distributed over 338 homesteads out of the 2,100 homesteads in the study area. The dataset included 514 child years of follow-up, with a mean incidence of 0.7 episodes of febrile malaria per child year and a prevalence of asymptomatic parasitaemia of 14%. Anopheles sporozoite rates and entomological inoculation rates A total of 284 light trap catches were conducted in a total of 150 houses, and 65% of the houses sampled had at least one Anopheles . 611 Anopheles mosquitoes were collected. Out of the 611 adult Anopheles mosquitoes caught, 480 were selected at random for PCR testing [21] . The species composition was 94.1% A. gambiae s.s. ( N =452), 3.54%, Anopheles arabiensis ( N =17), 1.25% Anopheles merus ( N =6) and 1.04% A. funestus ( N =5). All 611 samples were tested by ELISA for the P. falciparum circumsporozoite protein to detect sporozoites, and 1.47% (9/611) were positive (all of which were A. gambiae s.s.). Entomological inoculation rates (EIR) were calculated as previously described [21] . The overall EIR for the study area was 21.7 infective bites per person per year. Larval sites A total of 32 aquatic habitats were identified and sampled. The identified habitats consisted of stream pools (53.1%), pond-shores (34.4%), puddles (3%) and a dam. All the habitats had a muddy substrate and were semi-permanent except the dam, which is a permanent water body. Anopheles mosquito larvae were present in 50% ( N =16) of the habitats. A total of 168 Anopheles larvae were collected. The most abundant were first instar (59.5%, N =100) and second instar (27.4%, N =46) larvae compared with third (7.7%, N =13) and fourth (5.3%, N =9) instars. A total of 14 pupae were found in 3 habitats. Potential predators (nymphs) and competitors (tadpoles) were present in all the habitats. 25 Culex larvae were collected. All Anopheles larvae and all pupae were identified to the sibling species level using species-specific primers. Following A. gambiae species PCR on larvae, we identified 1.7% A. arabiensis ( N =3), 2.3% A. funestus ( N =4) and 96% A. gambiae s.s. ( N =168). Out of the 14 Pupae found, 85.71% ( N =12) were identified as A. gambiae s.s. and the remaining 2 that failed to amplify following PCR, by both A. gambiae and A. funestus species primers, were presumed to be Culex pupae. 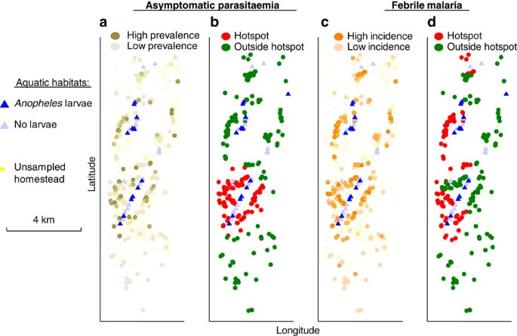Figure 1: Location of larval sites and homesteads showing malaria incidence. Plots of homesteads (circles) and larval sites (triangles) by longitude and latitude. (a) shows prevalence of asymptomatic parasitaemia by homestead, (b), hotspots of asymptomatic parasitaemia, (c), incidence of febrile malaria, and (d), hotspots of febrile malaria. Malaria infection Figure 1a,c shows the distribution of asymptomatic parasitaemia and febrile malaria, respectively, relative to the different larval sites. We used SaTScan to identify one hotspot of asymptomatic parasitaemia and three hotspots of febrile malaria ( Table 1 ; Fig. 1b,d ). The second most significant hotspot of febrile malaria partially overlapped the hotspot of asymptomatic parasitaemia. Figure 1: Location of larval sites and homesteads showing malaria incidence. Plots of homesteads (circles) and larval sites (triangles) by longitude and latitude. ( a ) shows prevalence of asymptomatic parasitaemia by homestead, ( b ), hotspots of asymptomatic parasitaemia, ( c ), incidence of febrile malaria, and ( d ), hotspots of febrile malaria. Full size image Table 1 Hotspot characteristics. Full size table Spatial relationship between malaria infection and larval sites The incidence of febrile malaria and prevalence of asymptomatic parasitaemia was associated with shorter distances from the homestead to the closest larval site ( Tables 2 and 3 ). However, the bearing at which the closest breeding site lay also determined risk. 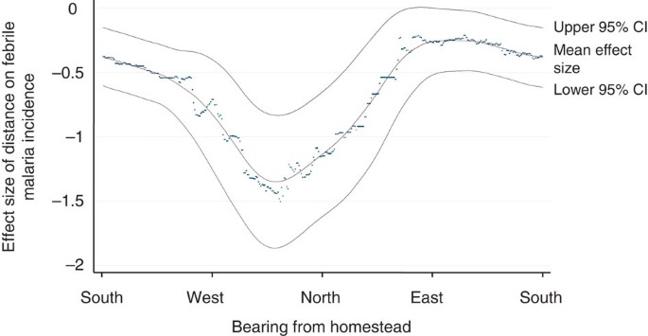Figure 2: Effect of bearing and distance between larval site and homestead on febrile malaria incidence. Each point on the graph is aggregated for a 180-degree arc of bearings, 90 degrees either side of the central direction indicated on theyaxis. Thexaxis indicates the effect size in a linear regression model of distance from breeding site on febrile malaria incidence. 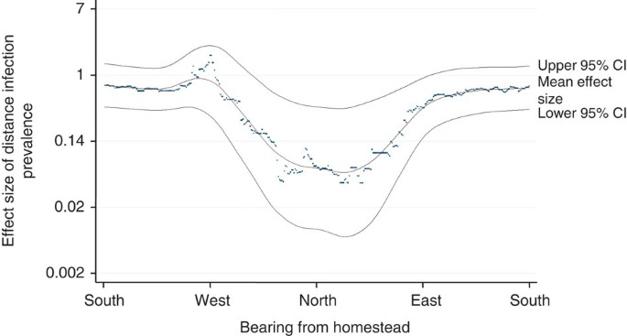Figure 3: Effect of bearing and distance between larval site and homestead on prevalence of asymptomatic parasitaemia. Each point on the graph is aggregated for a 180-degree arc of bearings, 90 degrees either side of the central direction indicated on theyaxis. Thexaxis indicates the odds ratio from a logistic regression model of distance from larval site on asymptomatic parasitaemia. The effect of bearing is demonstrated by the significant interactions between the vectors North or East and distance in determining risk of febrile malaria ( Table 2 ) and between the vector North and distance in determining the risk of asymptomatic malaria ( Table 3 ). These interactions are visualized in Figures 2 and 3 which show that the greatest effect size of distance in determining risk of febrile malaria or asymptomatic malaria occurred when the larval site lay in a northwesterly, or in a northerly direction, respectively. Table 2 Association of homestead and larval site variables and interactions with incidence of febrile malaria. Full size table Table 3 Association of homestead, larval site variables and interactions with prevalence of asymptomatic malaria. Full size table Figure 2: Effect of bearing and distance between larval site and homestead on febrile malaria incidence. Each point on the graph is aggregated for a 180-degree arc of bearings, 90 degrees either side of the central direction indicated on the y axis. The x axis indicates the effect size in a linear regression model of distance from breeding site on febrile malaria incidence. Full size image Figure 3: Effect of bearing and distance between larval site and homestead on prevalence of asymptomatic parasitaemia. Each point on the graph is aggregated for a 180-degree arc of bearings, 90 degrees either side of the central direction indicated on the y axis. The x axis indicates the odds ratio from a logistic regression model of distance from larval site on asymptomatic parasitaemia. Full size image Homestead distribution The number of homesteads along the line of flight between the larval site and the homestead reduced the risk of both febrile malaria and asymptomatic parasitaemia ( Tables 2 and 3 ), but this was not a factor after adjusting for distance (that is, the number of homesteads between the larval site, and homestead was simply a proxy for distance in this model). The population density immediately around the homestead was also associated with increasing risks of febrile malaria and asymptomatic parasitaemia but was not a factor after adjusting for distance from larval sites. Topography The altitude in the study area varied from 16-to-182 m above sea level. The ascents or descents along the line of flight between larval site and homestead did not influence risk ( Tables 2 and 3 ). The mean enhanced vegetation index (EVI) was similar throughout the study area, and so was not used further in analysis. Vegetation The mean EVI and seasonal maxima and minima did not vary throughout the study site, and was not used for further analysis. However, the variance of the waveform did vary substantially. There was no direct association between the variance of EVI and malaria risk ( Tables 2 and 3 ), but there was an interaction between the EVI variance along the line of flight between larval site and homestead and distance between the larval site and homestead. Multivariable models In a multivariable Poisson model using the significant ( P <0.05) predictors of febrile malaria from univariable analysis, two interaction terms remained independently significant: distance and northerly vector (incident rate ratio, IRR=0.54, 95%CI 0.33–0.88, P =0.015) and distance and EVI variance (IRR=0.84, 95%CI 0.74–0.96, P =0.008). In a multivariable logistic regression model to predict asymptomatic malaria, the interaction between distance and northerly vector remained significant (OR=0.18, 95%CI 0.04–0.8, P =0.024) and the interaction between distance and EVI variance was borderline (odds ratio, OR=0.72, 95%CI 0.51–1.02, P =0.063). We used a nearest neighbour method to test for spatial auto-correlation. Auto-correlation was significant for the first and second nearest neighbours (IRR=1.13, 95%CI 1.05–1.21, P <0.001 and IRR=1.19, 95%CI 1.14–1.25, P =0.001, respectively), but not for the third nearest neighbour (IRR=0.99, 95%CI 0.84–1.05, P =0.8). We therefore adjusted a multivariable model including first and second nearest neighbours as well as average age in the homestead (IRR=0.93 per year, 95%CI 0.86–1.00, P =0.06) and gender mix (IRR=1.18, 95%CI 0.89–1.57, P =0.26). After adjusting, the interactions between distance and northerly vector (IRR=0.46, 95%CI 0.26–0.82, P =0.008), and between distance and EVI variance (IRR=0.82, 95%CI 0.69–0.98, P =0.028) were similar to those observed without adjustment ( Table 2 ). Wind direction The prevailing wind direction measured at Mombasa airport was southerly 52% of the time and easterly 30% of the time. The mean north and east vectors were −0.37 (95%CI −0.40 to −0.34) and 0.30 (95%CI 0.27–0.32), respectively. When analysis was restricted to the hours between 21:00 and 9:00, the wind direction was southerly 63% of the time. 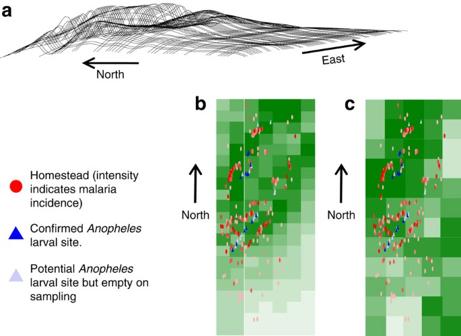Figure 4: Elevation and normalized vegetation index in the study area. Variation in elevation (a) and variance in normalized vegetation index with overlain homestead and larval site locations (b,c). When restricted to the rainy-season, wind direction was southerly 90% of the time ( Table 4 ). Table 4 Wind parameters by season and time of day. Full size table We also had access to data on wind direction in Kilifi Town, where observations are made once daily at midday. Out of the 104 observations made between 23 July 2010 and 3 November 2010, the wind was southerly 94% of the time and easterly for 6%. This study describes the association between spatial location of Anopheles larval sites and the occurrence of febrile and asymptomatic malaria in Junju, in Kilifi District on the Kenyan Coast. As in previous studies [16] , [17] , we found that the households located nearest to larval sites were at greater risk of malaria. This is as expected, because Anopheles mosquitoes have a limited dispersion distance [14] , [22] and are likely to seek a blood meal from the nearest household available. We have shown that the relationship between distance from a larval site and malaria risk is highly dependent on the direction of flight ( Figs 2 and 3 ). Where the larval site lies to the north or northwest of a homestead, proximity to the larval site and homestead has a strong effect on malaria infection. On the other hand, when the larval site lies to the south, proximity has little or no effect. This was not explained by topography, variations in the vegetation index or by surrounding population densities. However, the prevailing wind direction is southerly, and second most frequently easterly. This wind direction is not consistent with the land-/sea-breeze cycle, which would result in a westerly breeze during the early evening. However, the southerly trade wind is usually dominant during the rainy season [23] , as seen in our data. Mosquitoes identify human hosts at a distance by a variety of olfactory cues. Over shorter distances (for example, within the homestead), olfactory cues, host body temperature and CO 2 lead them to land on a host for a blood meal [24] . However, to identify the homestead in the first place requires them to trace odour through attraction to human volatiles from a distance [14] . Mosquitoes in the field have been observed flying both upwind [25] and downwind to identify hosts [26] . Our data is consistent with upwind searches in our study area, and we are the first to suggest that the prevailing wind can be used to predict the location of key larval sites relative to known malaria hotspots. A limitation of our study is that we did not have detailed data on local wind direction. One might expect local wind direction to be dominated by variable gusts of wind. Data on microvariation in local wind direction might explain further residual variation in malaria risk. Nevertheless, our data suggest that prevailing wind direction is strongly influential in determining malaria risk irrespective of the role of microvariations. A further limitation is that we relied on ground-searches and local resident's knowledge to identify larval sites. We examined for larval sites during the rains, in September 2010, and it is possible that some semi-permanent sites were present at other times, although the density of larval sites identified was consistent with previous studies in similar areas [27] . Asymptomatic parasitaemia was also assessed at a single time-point, and parasites may have been acquired many months previously. However, we have previously shown that the spatial heterogeneity, defined by asymptomatic parasitaemia, is stable over time, and furthermore that spatial heterogeneity in asymptomatic parasitaemia and febrile malaria does not seem to be strongly seasonal. [11] Taking this together with our finding that the combination of proximity to known site and direction of the site relative to prevailing wind is strongly predictive of malaria risk, we conclude that the relevant larval sites were identified in this study. Although proximity and direction of hosts from larval sites were strong correlates of malaria risk, as expected, there was substantial residual variation in malaria risk (pseudo r 2 =0.095). In Figure 1 , substantial variation in risk between homesteads in the clusters around hotspots can be identified, as can a few clusters of high incidence some distance from larval sites. However, this variation occurs at too fine a spatial scale to be readily explained by missed larval sites, and is poorly accounted for by autocorrelation (pseudo r 2 =0.02), suggesting that individual homestead factors may be responsible. Furthermore, factors such as homestead construction, varying behaviour patterns regarding bednet use, outdoor or indoor cooking, and socio-economic status may also determine risk, and these were not captured in our study. However, as the study participants were from a single ethnic group (that is, Chonyi) and relied entirely on subsistence farming in this area, it is unlikely that any of these factors were geographically clustered. The failure of larval habitats to produce high numbers of mature larvae and pupae has been described previously [28] . Early Anopheles larval instars are highly subject to predation, reducing the correlation between larval numbers and adult mosquito densities [28] . The presence of few large larvae or pupae might be taken to indicate that the larval sites that we identified were not producing adults. However, the most likely explanation of the strong correlations between distance from the larval sites and human malaria cases is the dispersion of adult mosquitoes, and so a more likely explanation is that the numbers of large larvae or pupae were few compared with earlier instars (owing to predation), and so not identified at a single assessment. Globally EIRs in the hundreds or even thousands have been reported [29] , but in the context of mass ITN distributions and generally falling transmission in Kilifi district [6] , an EIR of 21.7 is high. The EIR measurement represents an average for the study area and so is inadequate to reflect transmission intensity in the hotspots. However, if outdoor biting is significant, as has been observed in some areas of Kenya [30] , then the EIR that we measured based on indoor collections may be an underestimate. The topography along the presumed line of flight was not associated with altered risk (suggesting that, in this study area, flying uphill or downhill makes little difference to the mosquitoes), but there were interactions between the variance of the EVI along the line of flight and the distance travelled. Because the mean EVI throughout the study area was constant at the level of resolution available (that is, 0.25 km 2 ), we could not examine the effect of density of vegetation per se . Areas with a high variance of EVI are those that deviate from the usual seasonal pattern [31] . This may reflect use of the land for farming, or a type of vegetation more prone to seasonal variations in weather. The population in this study area are subsistence farmers, with a focus on maize crops (associated with seasonal variations), but there are also areas of dense coconut palms, which show less seasonal variation. It may be that mosquitoes found it harder to travel through areas with a high variance of EVI, as the interaction between variance of EVI and distance from larval site was in the direction of a lower risk of infection than would have been predicted by distance alone ( Tables 2 and 3 ). The EVI data and direction of travel both independently interacted with distance from the larval site, indicating that one did not confound the other. However, the EVI data was available at a resolution of 0.25 km 2 , and substantial variation in vegetation is likely to be present at a finer scale. Although 60% of the population used a bednet [32] , A. gambiae s.s. was still the most common vector. This contrasts observations in Western Kenya, where a shift in vector composition following increased use of long-lasting insecticidal nets, has been recently reported, and A. arabiensis is currently the primary vector of malaria [33] . Our demonstration that, on a fine scale, the heterogeneity of malaria risk is strongly related to identifiable larval sites in coastal Kenya suggests that targeted vector control may be an effective way of dealing with residual hotspots of transmission. Key larval sites are most likely to be found downwind from hotspots in coastal Kenya. The precise nature of the interaction between larval sites and wind direction in determining hotspots may be specific to our setting (that is, with a consistent night-time prevailing wind and with A. gambiae as the vector). However, malaria hotspots [8] , [34] , [35] , the association between malaria risk and proximity to larval sites [16] , [17] , and the influence of wind direction on mosquito flight [25] , [26] have been widely reported elsewhere in Africa. Hence, it is likely that wind direction has a substantial impact on the spatial epidemiology of malaria outside of coastal Kenya. Targeting hotspots is expected to be highly effective as a means of malaria control [12] . Hand searches for larval sites are labour intensive, but our data suggest that surveillance of malaria episodes may lead to the identification of key larval sites, where vector control could be targeted. Depending on the local vector ecology, this may be using larval control, targeted indoor residual spraying (IRS) or more novel vector control strategies [36] . Study location and human subjects The approval for human participation in this study was given by Kenya Medical Research Institute Scientific committee and National Review and Ethical Committee of Kenya Medical Research Institute, and was conducted according to the principles of the declaration of Helsinki. The study was conducted in a rural area on the coast of Kenya, namely Junju sublocation of Kilifi District (longitude 39.708–39.816 and latitudes −3.8978 to −3.7107). 642 children aged between 1 and 10 years old were recruited following written informed consent from their parents. Once recruited, follow-up continued even if children passed their 10th birthday during the study. Malaria surveillance was conducted for a full calendar year (that is, 2010), and larval sampling was conducted in September, during the rainy season. Surveillance for malaria The field methods used to identify episodes of febrile malaria and asymptomatic parasitaemia have previously been described [37] . Weekly active surveillance was undertaken, and children with fever had blood slides for malaria parasites taken. Blood smears were done only on children with an objective fever (that is, temp. ≥37.5 °C). On subjective fever, children were seen again 6–12 h later to repeat the temperature measurement. Blood smears were made if objective fever was confirmed at the later measurement. Trained field workers were available at all times in the villages for passive surveillance, and were present at the local dispensaries in the study area. Anti-malarials were supplied for proven episodes of malaria by the study team in accordance with government of Kenya guidelines (that is, Co-artemether). Study subjects may have used private clinics or bought anti-malarials without the study teams' knowledge, but given the all-hours access to free treatment via study staff, this was an unlikely occurrence. Surveys for asymptomatic parasitaemia were undertaken once during the year, immediately before the rainy season. All subjects recruited to the study were asked to attend for venous blood sampling, and thick-and-thin films were Giemsa-stained and examined by microscopy as per standard methods [38] . Results were available for 90% of the participants. The Geographic positioning system coordinates from the Kilifi demographic surveillance survey were linked to each homestead in the study. Definition of febrile malaria incidence and parasite rates Episodes of febrile malaria were determined using a parasite density threshold of >2,500 μl −1 (ref. 39 ). Multiple identifications of fever and parasitaemia within 21 days were considered a single episode. The incidence per homestead per year was calculated by episodes of febrile malaria per homestead, divided by the number of children and by the number of years that subjects were monitored. The parasite rate per homestead was calculated as the percentage of blood films positive for P. falciparum malaria from afebrile subjects at scheduled blood sampling. Adult mosquito catches and larval sampling Adult mosquitoes were sampled inside a total of 150 houses during the month of September 2010, and each house was sampled 2 times over a period of 15 days. CDC light traps were hung over the sleeping area and set overnight from 18:00 to 6:00. Adult mosquitoes were recovered from the traps each morning and identified to species using morphological keys. All anopheline mosquitoes were tested by enzyme-linked immunosorbent assay to determine sporozoite infection. A subset of Anopheles samples ( n =480, chosen at random but also including all those positive for sporozoites) were tested by PCR to determine A. gambiae and A. funestus sibling species. Our team of field workers conducted intensive ground searches to identify aquatic habitats that they sampled for mosquito larvae. In addition, they made enquiries from local residents regarding the location of stagnant water bodies in the area. Kilifi District is generally dry, with porous coral rock, and has a very limited piped water system. During the rainy season, residents often use water from stagnant pools for domestic use, despite many of these being temporary. Only one permanent site was identified, as a result of a dam, which was not productive of Anopheles larvae. Anopheles positive habitats were subsequently characterized based on type, appearance and size, and sampled for larvae using the 350-ml mosquito dippers (Bio-Quip Products). Larval habitat types were mainly stream pools, pond shores and puddles. Each habitat was surveyed for the presence of Anopheles larvae, which were sampled along the edge of each habitat using the standard dipping method. Larvae from each habitat were then transferred by pipetting into separate whirl-pak bags (Bio-Quip) and later sorted, counted and identified in the laboratory by morphology followed by species-specific PCR. For each larval habitat, longitude and latitude data were recorded using a handheld GPS (Garmin International). Analysis of hotspots The SaTScan software [40] was used to calculate the spatial scan statistic [41] . The spatial scan statistic uses a scanning window that moves across space. For each location and size of the window, the number of observed and expected cases is counted, and the window with the greatest ratio of observed-to-expected cases is noted. The scan statistic was then calculated for two types of cluster; to identify clusters (or 'hotspots') of febrile disease, using a discrete Poisson model; and to identify clusters (or 'hotspots') of asymptomatic parasitaemia, using a Bernoulli model, where cases were subjects with parasitaemia, and controls were subjects without parasitaemia. The test of significance was based on a Poisson-generalized likelihood ratio test, using 9,999 replications for a Monte-Carlo inference. The maximum cluster/hotspot size was set at 30% of the population, and the inference level for significance was set at 0.05 for primary clusters/hotspots. After removing the primary cluster/hotspot, the Scan statistic was recalculated for the remaining locations to identify secondary clusters/hotspots. Enhanced vegetation index and topographical data MODIS is a sensor on-board two NASA satellites. MODIS-derived temperature and reflectance layers were acquired for the years 2001 through 2008 (ref. 42 ). The EVI) was processed by a temporal Fourier algorithm to achieve temporal ordination of the data time series while preserving important aspects of seasonal variation in the measures [31] . The EVI was available in km square pixels. Topographical data was downloaded from Google Earth in 0.25 km square pixels. These pixels and related homestead locations are shown in Figure 4 . Figure 4: Elevation and normalized vegetation index in the study area. Variation in elevation ( a ) and variance in normalized vegetation index with overlain homestead and larval site locations ( b , c ). Full size image Meteorological data Data on wind direction and wind speed were recorded in Kilifi town, using a Sutron Hydromet Station, according to the manufacturer's instructions. The UK Meteorological Office supplied data from Mombasa airport. Model fitting to predict malaria risk Univariable and multivariable Poisson regression models were constructed to predict febrile malaria incidence, adjusting for child years of observation as an offset, and the following parameters as independent predictors: distance from larval sites, number of larvae in the nearest larval site, the vector of the direction in which the nearest larval site lay, the population density around the homestead, the population density between the larval site and the homestead, and the topographical profile between the larval site and the homestead. Because multiple individuals were present in homesteads, Poisson regression models were run to predict the risk of asymptomatic parasitaemia, considering the number of asymptomatic infections per homestead as the outcome. Interactions were examined using the product of two continuous independent variables, and significance testing done by comparing the interaction model with a fixed effects model using the log likelihood ratio test. How to cite this article: Midega, J.T. et al . Wind direction and proximity to larval sites determines malaria risk in Kilifi District in Kenya. Nat. Commun. 3:674 doi: 10.1038/ncomms1672 (2012).